Genomic analysis of ADAR1 binding and its involvement in multiple RNA processing pathways Adenosine deaminases acting on RNA (ADARs) are the primary factors underlying adenosine to inosine (A-to-I) editing in metazoans. Here we report the first global study of ADAR1–RNA interaction in human cells using CLIP-seq. A large number of CLIP sites are observed in Alu repeats, consistent with ADAR1’s function in RNA editing. Surprisingly, thousands of other CLIP sites are located in non- Alu regions, revealing functional and biophysical targets of ADAR1 in the regulation of alternative 3′ UTR usage and miRNA biogenesis. We observe that binding of ADAR1 to 3′ UTRs precludes binding by other factors, causing 3′ UTR lengthening. Similarly, ADAR1 interacts with DROSHA and DGCR8 in the nucleus and possibly out-competes DGCR8 in primary miRNA binding, which enhances mature miRNA expression. These functions are dependent on ADAR1’s editing activity, at least for a subset of targets. Our study unfolds a broad landscape of the functional roles of ADAR1. The proteins adenosine deaminases acting on RNA (ADARs) are known as the main mediators of adenosine to inosine (A-to-I) editing in metazoans [1] , [2] , [3] . Previous studies revealed ample evidence for the essential roles of ADAR proteins in life. Three ADAR family members have been identified in vertebrates: ADAR1 , ADAR2 and ADAR3 . The ADAR1 protein has two isoforms (long p150 and short p110) resulting from alternative promoters and start codons. The full-length ADAR1 p150 is induced by interferon, whereas ADAR1 p110 and ADAR2 are relatively ubiquitously expressed [4] , [5] . ADAR3, whose function remains unknown, was detected only in central nervous system [6] . Both ADAR1 and ADAR2 knockout (KO) mice showed severe phenotypes, with ADAR1 KO being embryonic lethal and ADAR2 KO surviving for only a few weeks after birth [7] , [8] . In C. elegans , ADAR mutants displayed deficiency in chemotaxis and longevity [9] , [10] . In addition, human ADAR mutations are associated with a number of diseases such as sporadic amyotrophic lateral sclerosis, the Aicardi–Goutieres syndrome and hepatocellular carcinoma [11] , [12] , [13] , [14] . Thus far, the main molecular function of ADAR1 and ADAR2 is known to be catalysis of A-to-I RNA editing. With double-stranded RNA (dsRNA)-binding domains (dsRBDs), these proteins recognize dsRNA structures, the best-known substrates for A-to-I editing. ADAR dsRBDs were generally assumed to bind nonspecifically to any dsRNA. However, recent studies revealed both sequence and structural characteristics that may determine preference or selectivity for deamination of particular adenosines among others [15] . Since the vast majority of human A-to-I editing sites are located in non-coding regions especially Alu elements [16] , [17] , [18] , it is believed that ADAR-binding sites should also be enriched in such regions, although this question has not been addressed on a genome-wide scale. In addition to RNA editing, ADAR proteins may affect other aspects of gene expression such as alternative splicing, miRNA biogenesis or targeting, mRNA decay and viral RNA degradation [3] , [19] , [20] . Indeed, following perturbation of cellular expression of ADARs, numerous alterations in the gene expression levels or transcript structures can be observed [21] . Such changes may have resulted from diverse regulatory mechanisms of gene expression that may account for the embryonic lethality in ADAR1 KO mice. However, it is not clear whether ADAR1 is directly or indirectly involved in the various mechanisms underlying the above molecular observations. A significant knowledge gap in our understanding of ADAR1 function is its genome-wide binding profile. To this end, we carried out the first global study of ADAR1 binding in human cells using the crosslinking immunoprecipitation (CLIP) method followed by high-throughput sequencing (CLIP-seq). Among the 23,782 reproducible ADAR1-binding sites in >10,000 protein-coding genes, the majority overlaps with Alu repeats, providing the first global confirmation of ADAR1’s preference for Alu s. However, a surprisingly large fraction (15%) of binding sites is located in non- Alu regions. While ADAR1 binding to Alu regions enables the discovery of new insights regarding A-to-I editing, its binding to non- Alu sites reveals a number of functional roles related to regulation of alternative 3′ untranslated region (UTR) usage and primary miRNA processing in the nucleus. Our study expands the landscape of the functional roles of ADAR1 that contributes to a better understanding of this essential protein. ADAR1 CLIP-seq in human cells To elucidate the function of ADAR1 on the genome-wide scale, we first obtained global binding patterns of this protein using CLIP-seq [22] in human U87MG cells. In this cell type, ADAR1 is expressed at a medium to high level, while ADAR2 and ADAR3 are barely expressed [21] . We constructed two libraries using two ADAR1 antibodies (Santa Cruz Biotechnologies). Both antibodies can recognize two isoforms of ADAR1 (p150 and p110) ( Supplementary Fig. 1 ). 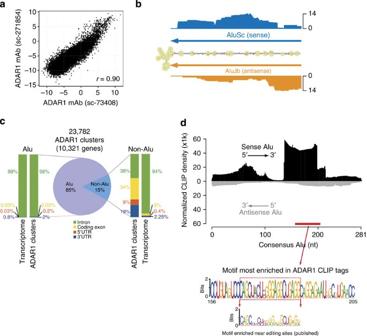Figure 1: CLIP-seq identifies ADAR1-binding sites in >10,000 human genes. (a) Reproducibility of ADAR1 CLIP tags using two different antibodies. Each dot in the scatter plot represents log2 enrichment relative to the background abundance measured by polyA+RNA-seq for a RefSeq transcript. (b) CLIP tag distribution in the 3′ UTR of thePSMBgene. The secondary structure of this region is shown as predicted by RNAfold. The number of CLIP tags is shown for each corresponding position in the folded structure, together with the location of twoAlusequences (inverted repeats). Known editing sites (DARNED database) are labelled with red dots. (c) Genomic distribution of reproducible ADAR1 CLIP sites. Similar distribution of nucleotides in the entire transcriptome is shown as a reference. (d) Alignment of CLIP reads to the consensusAlusequence. The CLIP tag density was normalized against expected tag density obtained from simulated reads to represent overall sequence enrichment of all the relevantAlus. Alignment to the senseAluconsensus and antisenseAluconsensus was carried out separately. Given their strand-specific nature, CLIP reads were aligned to either the sense or antisenseAluunambiguously. The motif most enriched in ADAR1 CLIP tags is shown (based on an independent motif search within CLIP clusters by Multiple Em for Motif Elicitation), which is located in the senseAluas labelled by the red bar. The motif enriched near editing sites in U87MG cells discovered previously21is also shown for comparison purpose. From each CLIP library, more than 10 million reads were obtained with confident mapping to the human genome ( Supplementary Table 1 ). To assess the reproducibility of the experiments, we examined the correlation of CLIP-seq tag abundance between the two libraries precipitated with different antibodies. As shown in Fig. 1a , the two libraries yielded highly correlated results, suggesting that most of the CLIP tags reflect the common pool of ADAR1-interacting RNAs. Figure 1: CLIP-seq identifies ADAR1-binding sites in >10,000 human genes. ( a ) Reproducibility of ADAR1 CLIP tags using two different antibodies. Each dot in the scatter plot represents log2 enrichment relative to the background abundance measured by polyA+RNA-seq for a RefSeq transcript. ( b ) CLIP tag distribution in the 3′ UTR of the PSMB gene. The secondary structure of this region is shown as predicted by RNAfold. The number of CLIP tags is shown for each corresponding position in the folded structure, together with the location of two Alu sequences (inverted repeats). Known editing sites (DARNED database) are labelled with red dots. ( c ) Genomic distribution of reproducible ADAR1 CLIP sites. Similar distribution of nucleotides in the entire transcriptome is shown as a reference. ( d ) Alignment of CLIP reads to the consensus Alu sequence. The CLIP tag density was normalized against expected tag density obtained from simulated reads to represent overall sequence enrichment of all the relevant Alus . Alignment to the sense Alu consensus and antisense Alu consensus was carried out separately. Given their strand-specific nature, CLIP reads were aligned to either the sense or antisense Alu unambiguously. The motif most enriched in ADAR1 CLIP tags is shown (based on an independent motif search within CLIP clusters by Multiple Em for Motif Elicitation), which is located in the sense Alu as labelled by the red bar. The motif enriched near editing sites in U87MG cells discovered previously [21] is also shown for comparison purpose. Full size image One of the known types of ADAR1 substrate is the long dsRNA structure, such as the structure found in PSMB pre-mRNA [23] ( Fig. 1b ). As expected, we detected CLIP tags supporting ADAR1 binding to this dsRNA, most of which overlapped with the Alu elements. Furthermore, the binding sites of ADAR1 coincided with known RNA-editing sites in this region ( Fig. 1b ). To provide independent validation, we randomly picked examples of ADAR1-binding targets based on the CLIP-seq data and validated via traditional IP experiment followed by reverse transcription-PCR (RT–PCR; Supplementary Fig. 2a ). We chose these examples to cover the categories of LINE, Alu and 7SK RNAs, and was able to confirm ADAR1 binding to all of them. Together these results support the validity of our CLIP experiments. Transcriptome-wide-binding locations of ADAR1 Among all CLIP reads mapped to the human genome, the majority (~83%) resided in transcribed regions annotated by RefSeq. To identify ADAR1-binding locations distinguished from background noise in intragenic regions, we defined CLIP clusters by controlling for gene-specific background [24] . These ADAR1 CLIP-binding sites were generally uncorrelated with CLIP sites for other RNA-binding proteins (RBPs) for which data were publicly available, supporting the specificity of each CLIP data set ( Supplementary Fig. 2b ). However, we observed a small number of CLIP sites that appeared to be shared by multiple RBPs (for example, 2,461 clusters shared by at least three RBPs including ADAR1). This observation may suggest existence of functional interaction of these proteins. However, it may also reflect minor artifacts in CLIP due to non-protein-specific properties of the method in general. To be conservative, we filtered the ADAR1 CLIP clusters by removing common sites between ADAR1 and at least two other RBPs. Despite a possible loss of certain biological interactions, we applied this filter to enrich for sites that are predominantly related to ADAR1 itself. CLIP using the two antibodies generated 128,852 (sc-73408) and 53,715 (sc-271854) clusters, respectively, among which 32,876 (25.5% and 61.2%, respectively, for the two experiments) are common ( Supplementary Fig. 3 ). The common clusters were further filtered as described above resulting in 23,782 (in 10,321 genes) final clusters. For all the analyses below related to CLIP clusters, we used only clusters (or sites) that were common to both antibodies (unless noted otherwise) ( Supplementary Data 1 ). The first evident observation was that the majority of CLIP sites were located in Alu elements in introns ( Fig. 1c ), which is consistent with the known fact that most human A-to-I editing sites reside in Alus . ADAR1 binding to Alus was relatively depleted in coding exons, consistent with the known low abundance of A-to-I editing sites in coding regions. A surprisingly large fraction (15%) of ADAR1 sites was located in non- Alu regions. Intriguingly, these non- Alu sites were more enriched in coding exons and UTRs compared with the background consisting of the entire transcriptome ( Fig. 1c ). Among non- Alu sites, about 10 and 8% were mapped to LINE and other SINE repeats, respectively, consistent with recent findings that a small fraction of A-to-I editing occurs in such repeats [25] . However, the majority (75%) of non- Alu sites resided in non-repetitive regions. Binding preference of ADAR1 within Alu elements Despite the long-existing assumption of ADAR1 binding to Alu elements, it is not clear whether certain subregions of the repeats are preferably recognized by ADAR1 or ADAR1 binding has no preference within the repeats (structural or sequence-wise). The CLIP data allowed a detailed examination of this question. We realigned the mapped CLIP reads to the sense and antisense Alu consensus sequences and carried out an assessment of regional bias of read density. Such direct alignment to the consensus sequences also helps to avoid the problem of non-unique mapping. The CLIP density was then normalized against Alu -simulated tag density (Methods) to control for inherent sequence bias in Alu elements. As a result, strong enrichment of reads was observed near the right arm of the sense Alu ( Fig. 1d ). As an independent test of ADAR1-binding preference, we searched for sequence motifs enriched in the CLIP clusters with background controls generated by random Alu sequences. The most significant motif was located within the Alu consensus where high CLIP tag density was observed as shown in Fig. 1d . This result further attests to the existence of subregions in the Alu repeats preferred by ADAR1. Remarkably, the motif represents an extended version of the same motif that we previously discovered around A-to-I editing sites in U87MG cells [21] ( Fig. 1d ). It can form a palindromic secondary structure ( Supplementary Fig. 4 ), thereby likely reflecting the known dsRNA-binding property of ADAR1 rather than a sequence preference. Alternatively, it may represent a subsequence of extended binding regions of ADAR1 dimers [26] (for example, consisting of sense and antisense Alu pairs). Note that this motif is different from those identified near editing sites in Drosophila [27] , possibly due to the vast divergence of Alu -like sequences between human and Drosophila . We further observed that the motif, although enriched in ADAR1 binding sites, is not adequate to enable ADAR1 binding by itself ( Supplementary Fig. 5 ). Thus, future work is necessary to examine the functional relevance of this motif in ADAR1 editing. ADAR1 binding to Alus is closely related to RNA editing We next examined the relationship between ADAR1 binding and RNA editing in detail with a focus on CLIP sites within Alu repeats. We analysed the distance between ADAR1 CLIP clusters and their respective closest known A-to-I editing sites. As shown in Fig. 2a , the linear distance from binding to editing sites was significantly smaller than to controls calculated for random A’s in the same region. Moreover, the binding sites were even closer to editing sites if the distances were calculated between the editing sites and predicted dsRNA structures harbouring the CLIP cluster. In particular, >20% of Alu -containing structures overlapped with A-to-I editing sites and about 50% of the CLIP clusters were located relative to editing sites in a distance of at least two orders of magnitude closer than expected by chance. It should be noted that the absolute distance between CLIP clusters and editing sites is relatively high (median ~1 kb for the structured ones) possibly due to the facts that many more editing site are yet to be identified and/or the CLIP experiments did not capture all ADAR1-binding sites. 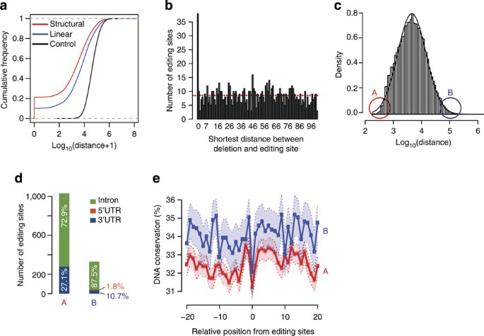Figure 2: ADAR1 binding signature reflects its function in RNA editing. (a) Shortest distance between ADAR1-boundAlusites and RNA-editing sites (DARNED database, same below) in the same gene. Linear: linear genomic distance; structural: distance calculated between predicted dsRNA structures harbouring the CLIP cluster and editing sites; control: distance between CLIP clusters and random A’s chosen from the same region as authentic editing sites. Both linear and structural distances are significantly smaller than control (P<2.2e−16, Kolmogorov–Smirnov test). (b) Histogram of distance (up to 100 nt) between deletions in CLIP reads and closest RNA editing sites in the same gene. Red dashed line represents the average distance in the range shown. (c) Histogram of closest distance between ADAR1-boundAluclusters in the same gene. A and B denote the bottom and top 5% of distances respectively. (d) Genomic distribution of editing sites within 100 nt ofAluclusters in groups A and B as defined inc. The distribution of these editing sites in different regions of annotated genes is shown. Note that no editing sites were found in coding exons. (e) Conservation level of positions surrounding editing sites in groups A and B across primates. DNA conservation was calculated as % sequence identify. Light-shaded area represents confidence intervals. Figure 2: ADAR1 binding signature reflects its function in RNA editing. ( a ) Shortest distance between ADAR1-bound Alu sites and RNA-editing sites (DARNED database, same below) in the same gene. Linear: linear genomic distance; structural: distance calculated between predicted dsRNA structures harbouring the CLIP cluster and editing sites; control: distance between CLIP clusters and random A’s chosen from the same region as authentic editing sites. Both linear and structural distances are significantly smaller than control ( P <2.2e−16, Kolmogorov–Smirnov test). ( b ) Histogram of distance (up to 100 nt) between deletions in CLIP reads and closest RNA editing sites in the same gene. Red dashed line represents the average distance in the range shown. ( c ) Histogram of closest distance between ADAR1-bound Alu clusters in the same gene. A and B denote the bottom and top 5% of distances respectively. ( d ) Genomic distribution of editing sites within 100 nt of Alu clusters in groups A and B as defined in c . The distribution of these editing sites in different regions of annotated genes is shown. Note that no editing sites were found in coding exons. ( e ) Conservation level of positions surrounding editing sites in groups A and B across primates. DNA conservation was calculated as % sequence identify. Light-shaded area represents confidence intervals. Full size image Some of the CLIP reads contained one or more deletions that corresponded to the crosslinking sites between the protein and the RNA [28] ( Supplementary Fig. 6 ). We further analysed the distance between such deletions and the nearest editing sites. Interestingly, a number of deletion sites coincided exactly with A-to-I editing sites, the observed frequency of which represented a greater than fourfold enrichment compared with random expectation ( Fig. 2b ). Thus, there is concordance between ADAR1–RNA crosslinking sites and deamination sites. This observation is consistent with a model where the deaminase domain comes to close proximity of the RNA to facilitate enzymatic reaction [29] , [30] . In addition, the precise capture of the deamination sites in CLIP supports the validity of our experiments. The distance between adjacent ADAR1-bound Alu sites varied in a considerable range spanning three orders of magnitudes ( Fig. 2c ). We asked whether this distance reflected certain structural difference among ADAR1 substrates as it is known that there exist two nominal types of ADAR1 substrates [31] . Long dsRNA structures are often associated with hyperediting (promiscuous), whereas short structures showed site-selective editing. Thus, we focused on the two groups located at the two extremes of the distance distribution ( Fig. 2c ) to maximize the possible difference to be observed. In the first group (group A), multiple Alu sites were located in close proximity, which may constitute a single long dsRNA structure. The second group (B) containing singleton Alu site far away from other CLIP sites may form short stem-loop structures by itself. Since the prediction of RNA secondary structures is not yet accurate, we focused on analysing the features of RNA editing in the two groups. Interestingly, for groups A and B, there existed a striking difference in the enrichment of RNA editing sites in the neighbourhoods of the CLIP clusters. As shown in Fig. 2d , group A had much more editing sites than group B, with both classes of editing sites preferentially located in introns or 3′ UTRs. In addition, group B editing sites resided in regions with higher DNA sequence conservation than editing sites in A ( Fig. 2e ). Thus, it is likely that group A is enriched with substrates for hyperediting (promiscuous) and group B corresponds to site-selective editing that are known to be under enhanced evolutionary selection [31] . ADAR1 binding to non- Alu regions affects 3′ UTR usage Given the enrichment of non- Alu sites in 3′ UTRs ( Fig. 1c ), we next investigated whether ADAR1 affects the formation of 3′ UTRs. We first conducted a genome-wide analysis of 3′ UTR length in U87MG cells using RNA-seq data obtained following ADAR1 knockdown (KD) or control siRNA transfection [21] . Following a customized 3′ UTR analysis in RNA-seq (Methods), we extracted expression levels of the core and extension regions of 3′ UTRs with alternative forms resulted from alternative polyadenylation (APA). Many 3′ UTRs were identified with altered expression in the core or extension regions ( Fig. 3a ), four randomly chosen examples of which were confirmed in experimental validation ( Fig. 3b , Supplementary Fig. 7 , and Supplementary Table 2 ). 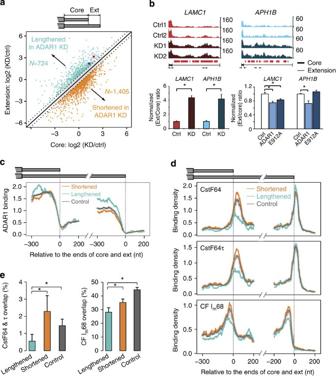Figure 3: ADAR1 is involved in the regulation of alternative 3′ UTR usage. (a) Expression levels of core and extended (ext) regions of tandem 3′ UTRs identified in RNA-seq data. Scatter plot of their expression change following ADAR1 KD in U87MG cells compared with control siRNA transfection is shown. Those with at least 41.4% change (log2-fold-change >0.5) are marked with colours. Two groups are labelled: UTRs that were lengthened in ADAR1 KD cells and the opposite. The number of 3′ UTRs in each group is shown. (b) Examples of ADAR1-regulated 3′ UTRs (with the two genes labelled as big red and blue dots ina). Read distribution plots in two biological replicates of RNA-seq of control (Ctrl) and ADAR1 KD experiments are shown. To compare the relative coverage of extension and core regions, read counts were normalized such that the maximum count of the core region of each gene is the same in the four samples. Locations covered with CLIP reads are denoted as small red bars below the RNA-seq read distribution. Real-time PCR validation is shown with primers illustrated as small arrows (primers within core regions are enlarged in the illustration due to limited core length). Expression of extension regions was normalized by that of the core region. The ratios were further normalized such that controls have a value of 1. Mean±s.d. is shown for six biological replicates. *P<0.05 (Wilcoxon rank-sum test). (c) Mean ADAR1 CLIP density near the 3′ end of core and extension regions in the two groups as defined ina. CLIP density was normalized using gene expression levels (RPKMs) derived from RNA-seq data. Similarly normalized density in control 3′ UTRs is shown. The controls (grey dots ina) were randomly picked to match the RPKM values of the regulated 3′ UTRs. Confidence intervals (95%) are shown for the control curves that were calculated using 100 sets of randomly constructed, RPKM matched controls. (d) Mean CLIP density near the 3′ end of core and extension regions of the same 3′ UTR groups as inc. The density was normalized in the same way as described inc. The controls were again randomly picked to match the RPKM values of the regulated 3′ UTRs. RNA-seq data of HEK 293 cells (same cell type as for the CLIP data shown here) were used to calculate gene-level RPKM. (e) Percent overlap between ADAR1 targets and targets of the CstF64 and τ and CFIm68 calculated relative to the number of ADAR1 targets in the ‘lengthened’, ‘shortened’ (as defined ina) and controls (grey dots ina).Pvalues (*P<0.05) were calculated by proportion tests and the error bars show the 95% confidence intervals. The number of samples in each group is illustrated ina. Figure 3: ADAR1 is involved in the regulation of alternative 3′ UTR usage. ( a ) Expression levels of core and extended (ext) regions of tandem 3′ UTRs identified in RNA-seq data. Scatter plot of their expression change following ADAR1 KD in U87MG cells compared with control siRNA transfection is shown. Those with at least 41.4% change (log2-fold-change >0.5) are marked with colours. Two groups are labelled: UTRs that were lengthened in ADAR1 KD cells and the opposite. The number of 3′ UTRs in each group is shown. ( b ) Examples of ADAR1-regulated 3′ UTRs (with the two genes labelled as big red and blue dots in a ). Read distribution plots in two biological replicates of RNA-seq of control (Ctrl) and ADAR1 KD experiments are shown. To compare the relative coverage of extension and core regions, read counts were normalized such that the maximum count of the core region of each gene is the same in the four samples. Locations covered with CLIP reads are denoted as small red bars below the RNA-seq read distribution. Real-time PCR validation is shown with primers illustrated as small arrows (primers within core regions are enlarged in the illustration due to limited core length). Expression of extension regions was normalized by that of the core region. The ratios were further normalized such that controls have a value of 1. Mean±s.d. is shown for six biological replicates. * P <0.05 (Wilcoxon rank-sum test). ( c ) Mean ADAR1 CLIP density near the 3′ end of core and extension regions in the two groups as defined in a . CLIP density was normalized using gene expression levels (RPKMs) derived from RNA-seq data. Similarly normalized density in control 3′ UTRs is shown. The controls (grey dots in a ) were randomly picked to match the RPKM values of the regulated 3′ UTRs. Confidence intervals (95%) are shown for the control curves that were calculated using 100 sets of randomly constructed, RPKM matched controls. ( d ) Mean CLIP density near the 3′ end of core and extension regions of the same 3′ UTR groups as in c . The density was normalized in the same way as described in c . The controls were again randomly picked to match the RPKM values of the regulated 3′ UTRs. RNA-seq data of HEK 293 cells (same cell type as for the CLIP data shown here) were used to calculate gene-level RPKM. ( e ) Percent overlap between ADAR1 targets and targets of the CstF64 and τ and CFI m 68 calculated relative to the number of ADAR1 targets in the ‘lengthened’, ‘shortened’ (as defined in a ) and controls (grey dots in a ). P values (* P <0.05) were calculated by proportion tests and the error bars show the 95% confidence intervals. The number of samples in each group is illustrated in a . Full size image Alterations in 3′ UTR length following ADAR1 KD could reflect both direct and indirect effects of this protein. Indeed, a number of canonical cleavage and polyadenylation factors had altered transcript levels following ADAR1 KD ( Supplementary Table 3 ). In this work, we focus on the direct function of ADAR1 by incorporating protein–RNA-binding analysis. Compared with those unaffected by ADAR1 (controls), 3′ UTRs lengthened in ADAR1 KD (referred to as ‘lengthened’ 3′ UTRs henceforth) were enriched with ADAR1 CLIP sites in both core and extension regions ( Fig. 3c ). Such a difference was not observed for 3′ UTRs that expressed the shorter form following ADAR1 KD (that is, ‘shortened’ 3′ UTRs). The binding profile of ADAR1 in the 3′ UTRs showed broad peaks in the core and extension regions. In addition, the majority (83%) of CLIP sites in 3′ UTRs with length change fell into non- Alu regions, confirming that ADAR1 regulates alternative 3′ UTRs primarily through binding to non- Alu sites. In this study, we will focus on the lengthened 3′ UTRs since they are direct candidate targets of ADAR1. ADAR1 competes with known 3′ UTR-binding factors To shed light on the mechanistic role of ADAR1 in this process, we analysed the genomic signatures of known cleavage and polyadenylation-relevant proteins with respect to ADAR1-regulated 3′ UTRs. Using CLIP-seq data of a panel of proteins in the families of CF I m , CPSF, CstF and Fip1 (ref. 32 ), we observed considerable binding differences of CstF64, CstF64τ and CF I m 68 in 3′ UTRs affected by ADAR1 compared with controls ( Fig. 3d ). Specifically, there was a reduction in binding density of all three proteins flanking the proximal cleavage sites of lengthened 3′ UTRs. CF Im68 also demonstrated reduced binding upstream of the distal sites of these 3′ UTRs, although to a smaller extent. As indirect targets of ADAR1, shortened 3′ UTRs were observed with similar CstF64, CstF64τ and CF I m 68 binding profiles as controls. Thus, the shortened 3′ UTRs also serve as negative controls for the lengthened 3′ UTRs that are likely direct targets of ADAR1. Other proteins with CLIP data available [32] did not demonstrate significant differential binding in this analysis ( Supplementary Fig. 8 ). The above binding patterns motivated a hypothesis that ADAR1-regulated 3′ UTRs are less frequently bound, thus less regulated by CstF64, CstF64τ and CF I m 68 compared with control UTRs. We thus examined expression patterns of these 3′ UTRs in cells with reduced levels of the proteins [32] , [33] . Compared with control cells, cells with CF I m 68 KD were previously reported to exhibit global 3′ UTR shortening [32] , which is confirmed in our analysis for the group of control 3′ UTRs unaffected by ADAR1 ( Supplementary Fig. 9a ). In contrast, 3′ UTRs lengthened in ADAR1 KD showed less shortening compared with controls in CF I m 68 KD, supporting the hypothesis that CF I m 68 has less influence on these UTRs. Opposite to CF I m 68, the proteins CstF64 and CstF64τ are known to enhance usage of proximal cleavage sites, thus associated with global 3′ UTR lengthening in KD cells [33] . Since the two proteins are known to have redundant function, we analysed double KD data where both proteins had reduced expression [33] . As expected, we observed a bias towards lengthening of the control 3′ UTRs in double KD cells ( Supplementary Fig. 9b ). In contrast, the 3′ UTRs lengthened in ADAR1 KD showed less lengthening compared with controls in these cells (although the P value was not significant, possibly due to small sample size, Kolmogorov–Smirnov test). Consistent with the above data, we also observed that lengthened 3′ UTRs in ADAR1 KD had significantly less overlap with target 3′ UTRs previously reported for CstF64 (ref. 33 ) or CF I m 68 (ref. 32 ) compared with controls or the shortened group ( Fig. 3e ). Our results support the hypothesis that ADAR1-regulated 3′ UTRs are less often affected by the CF I m 68 and CstF64 proteins in the presence of ADAR1. One possible model is that ADAR1’s binding to the 3′ UTR regions precludes binding of other proteins. Motif analysis in search of binding sites of CF I m 68 and CstF64 (ref. 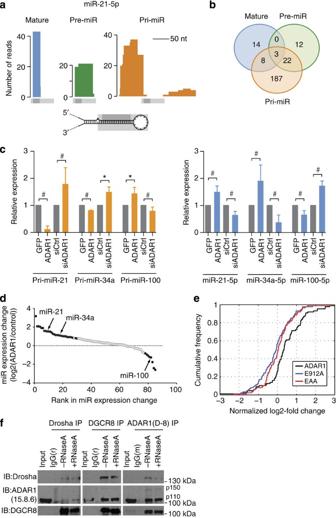Figure 4: ADAR1 mediates pri-miRNA processing. (a) CLIP reads mapped to the mature, precursor and primary transcripts of miR-21-5p. Light and dark grey bars represent the relative locations of annotated mature and pre-miR-21. Stem-loop structure is shown for illustration purpose only that does not reflect the true structure of pre-miR-21. (b) Numbers of mature, pre-miR and pri-miR bound by ADAR1 and numbers of miRNAs with two or three forms bound by ADAR1 (shown as overlaps). OverlapPvalues between pri-miR and pre-miR: 0.024, between pri-miR and mature: 0.79 and between pre-miR and mature: 0.18, calculated using hypergeometric test and assuming a total of 410 miRNAs being expressed in U87MG cells (based on small RNA-sequencing data). (c) Pri- (left panel) and mature miRNA expression (right panel) of endogenous miR-21-5p, miR-34a-5p and miR-100-5p in U87MG cells as measured by RT-qPCR. Cells were transfected with the pEGFP-C1 vector (GFP), pEGFP-C1-ADAR1 vector (ADAR1), scrambled siRNA (siCtrl) or siRNA for ADAR1 (siADAR1). Results (mean and s.d.) from ≥ four biological replicates are shown.#P<0.01, *P<0.05 (Wilcoxon Rank-Sum test). (d) Expression change of miRNAs in U87MG cells with ADAR1 perturbation (KD or OE) relative to controls. Only miRNAs whose primary transcripts were associated with ADAR1 CLIP reads are included. Filled circles represent miRNAs with significantly altered expression in KD or OE. If the significance was observed in both experiments or if no significance was found in either experiment, the average expression change is shown. If only one experiment led to a significant change, the value of expression change in this experiment is shown. Two miRNAs were excluded because they demonstrated significant changes in both experiments, but in conflicting directions. (e) Cumulative distribution functions of log2-fold changes (LFCs) of miRNAs bound by ADAR1 in the primary form in U87MG cells following OE of wild-type ADAR1, E912A or EAA mutants, compared with controls. The LFC values represent log2(OE/ctrls) that were further normalized by spike-in controls to account for technical variations across experiments. (f) ADAR1 associates with both DROSHA and DGCR8. Co-IP experiments were performed using DROSHA antibody (ab12286), DGCR8 antibody (ab90579), ADAR1 antibody (D-8) or corresponding rabbit (r) or mouse (m) isotype IgG in HeLa cells. HeLa cells were used since DROSHA and DGCR8 expression is relatively higher in HeLa than in U87MG cells. IP samples were immunoblotted (IB) using ADAR1 antibody (15.8.6), DROSHA antibody (ab12286) and DGCR8 antibody (ab90579) to detect the corresponding antigens. ADAR1 interacts with both DROSHA and DGCR8, reciprocally but not the corresponding IgG isotype control. RNase A treatment does not significantly impair the interactions. 32 ) around the proximal and distal cleavage sites did not yield significant difference in their enrichment in ADAR1-regulated 3′ UTRs versus controls ( Supplementary Table 4 ). Thus, it is likely that CF I m 68 and CstF64 can gain increased access to the ADAR1-regulated 3′ UTRs in cells with ADAR1 KD compared with control cells. The lengthening of these 3′ UTRs in ADAR1 KD cells could be resulted from a combinatorial function of multiple proteins, likely dominated by CF I m 68 that was reported to strongly enhance usage of distal cleavage sites [32] . Editing dependency of ADAR1-regulated 3′ UTR usage Binding of ADAR1 to 3′ UTRs can induce A-to-I editing. Thus, a related question is whether RNA editing is necessary to induce the observed influence of ADAR1 on 3′ UTRs. As expected, 3′ UTRs lengthened following ADAR1 KD showed enhanced occurrence of editing sites than other groups in regions where increased ADAR1 binding was observed ( Supplementary Fig. 10 ). However, only about 25% of these 3′ UTRs harbour at least one known A-to-I editing site [34] overlapping or close to the 3′ UTRs (±500 nt). Thus, we hypothesized that editing may contribute to ADAR1’s regulation of some, but not all 3′ UTRs. To test this hypothesis, we overexpressed an E912A mutant of ADAR1 that has an inactive deaminase domain [29] in U87MG cells. Overexpression of the wild-type ADAR1 or a control vector was carried out for comparisons. As shown in Fig. 3b , E912A overexpression abolished the 3′ UTR change observed for the wild-type ADAR1 for the gene APH1B , but not for LAMC1 . Note that APH1B has known A-to-I editing sites in the upstream intron of the 3′ UTR, but LAMC1 has no known editing sites close to the 3′ UTR. Thus, the impact of ADAR1 on 3′ UTR usage is dependent on RNA editing for some 3′ UTRs, but others could be affected by ADAR1 in an editing-independent manner. 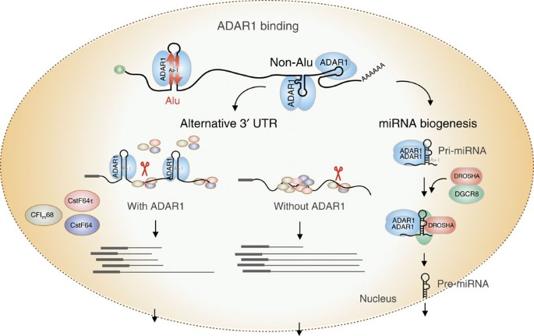Figure 5: Schematic models of ADAR1 function in the nucleus on 3′ UTR processing and miRNA biogenesis. These regulatory mechanisms are mainly executed by ADAR1 binding to non-Aluregions. ADAR1 may compete with other cleavage and polyadenylation factors (CF Im68, CstF64 and CstF64τ) in binding to 3′ UTRs. In the presence of ADAR1, the three proteins impose reduced regulatory influence on ADAR1-bound 3′ UTRs than on other 3′ UTRs. Following ADAR1 KD, these proteins could gain more access to the 3′ UTRs and exert regulation. The proximal cleavage site is often chosen in the presence of ADAR1, whereas the distal site is used on ADAR1 KD. These outcomes reflect combinatorial regulation by the cleavage and polyadenylation factors that have opposing impacts on alternative 3′ UTR usage. For pri-miRNA processing, ADAR1 may bind to (and edit) the nascent primary transcript before DROSHA/DGCR8 binding. The microprocessor then cleaves the pri-miRNA with or without binding to the RNA. The binding of ADAR1 mainly promotes the processing of pri-miRNA, leading to an enhanced miRNA expression level. Functional relevance of ADAR1-regulated 3′ UTR usage Gene ontology (GO) analysis of genes with 3′ UTR lengthening following ADAR1 KD showed enrichment of processes related to development and differentiation ( Supplementary Table 5 ). In addition, the genes involved in transcriptional regulation or metabolic processes were also enriched. For example, two of the SMAD family genes, SMAD1 and SMAD9 , were identified in this analysis. The SMAD proteins, as part of the transforming growth factor beta pathway, transduce extracellular signals to the nucleus and activate downstream gene transcription [35] . They contribute to important processes such as cellular growth, differentiation, apoptosis and development. Another protein, BRCA2, is involved in DNA damage repair through binding to single-stranded DNA and interacting with the recombinase RAD51 to stimulate homologous recombination [36] . In addition to breast cancer, this gene was also shown as a high-risk prostate cancer susceptibility gene [37] . Overall, our results suggest that ADAR1’s impact on APA could have significant functional implications, which should be further investigated in the future. ADAR1 binds to non- Alu regions harbouring pri-miRNAs In addition to coding genes, ADAR1 also interacts with non-coding RNAs within non- Alu regions, particularly miRNA transcripts, most of which do not overlap with Alu repeats. Our CLIP data allowed a genome-wide analysis of the interactions between ADAR1 and miRNA transcripts. We observed that ADAR1 could bind to all the three forms of miRNAs: primary (pri-), precursor (pre-) and mature miRNAs (Methods), an example of which is shown in Fig. 4a . Overall, 220, 37 and 25 pri-, pre- and mature miRNAs were associated with ADAR1, respectively ( Fig. 4b and Supplementary Table 6 ). Among the three forms of miRNAs, pri-miRNAs were most often observed with ADAR1 binding, possibly due to their longer length and/or the relative abundance of ADAR1 in the nucleus of U87MG cells ( Supplementary Fig. 11 ). A few miRNAs previously reported to be edited by ADAR1 (refs 38 , 39 ) were present in the ADAR1 CLIP primary miRNA list ( Supplementary Table 6 ), supporting our observed interactions between ADAR1 and primary miRNAs. Interestingly, 25 miRNAs were associated with ADAR1 in both precursor and primary transcripts, which is a significant overlap ( P =0.02, hypergeometric test; Fig. 4b ). These data together prompted the hypothesis that ADAR1 may affect pri-miRNA processing through interaction with the primary transcripts. Figure 4: ADAR1 mediates pri-miRNA processing. ( a ) CLIP reads mapped to the mature, precursor and primary transcripts of miR-21-5p. Light and dark grey bars represent the relative locations of annotated mature and pre-miR-21. Stem-loop structure is shown for illustration purpose only that does not reflect the true structure of pre-miR-21. ( b ) Numbers of mature, pre-miR and pri-miR bound by ADAR1 and numbers of miRNAs with two or three forms bound by ADAR1 (shown as overlaps). Overlap P values between pri-miR and pre-miR: 0.024, between pri-miR and mature: 0.79 and between pre-miR and mature: 0.18, calculated using hypergeometric test and assuming a total of 410 miRNAs being expressed in U87MG cells (based on small RNA-sequencing data). ( c ) Pri- (left panel) and mature miRNA expression (right panel) of endogenous miR-21-5p, miR-34a-5p and miR-100-5p in U87MG cells as measured by RT-qPCR. Cells were transfected with the pEGFP-C1 vector (GFP), pEGFP-C1-ADAR1 vector (ADAR1), scrambled siRNA (siCtrl) or siRNA for ADAR1 (siADAR1). Results (mean and s.d.) from ≥ four biological replicates are shown. # P <0.01, * P <0.05 (Wilcoxon Rank-Sum test). ( d ) Expression change of miRNAs in U87MG cells with ADAR1 perturbation (KD or OE) relative to controls. Only miRNAs whose primary transcripts were associated with ADAR1 CLIP reads are included. Filled circles represent miRNAs with significantly altered expression in KD or OE. If the significance was observed in both experiments or if no significance was found in either experiment, the average expression change is shown. If only one experiment led to a significant change, the value of expression change in this experiment is shown. Two miRNAs were excluded because they demonstrated significant changes in both experiments, but in conflicting directions. ( e ) Cumulative distribution functions of log2-fold changes (LFCs) of miRNAs bound by ADAR1 in the primary form in U87MG cells following OE of wild-type ADAR1, E912A or EAA mutants, compared with controls. The LFC values represent log2(OE/ctrls) that were further normalized by spike-in controls to account for technical variations across experiments. ( f ) ADAR1 associates with both DROSHA and DGCR8. Co-IP experiments were performed using DROSHA antibody (ab12286), DGCR8 antibody (ab90579), ADAR1 antibody (D-8) or corresponding rabbit (r) or mouse (m) isotype IgG in HeLa cells. HeLa cells were used since DROSHA and DGCR8 expression is relatively higher in HeLa than in U87MG cells. IP samples were immunoblotted (IB) using ADAR1 antibody (15.8.6), DROSHA antibody (ab12286) and DGCR8 antibody (ab90579) to detect the corresponding antigens. ADAR1 interacts with both DROSHA and DGCR8, reciprocally but not the corresponding IgG isotype control. RNase A treatment does not significantly impair the interactions. Full size image ADAR1 binding to pri-miRNAs alters miRNA expression We next examined the impact of ADAR1 on pri-miRNA processing of three example miRNAs whose primary transcripts were observed in ADAR1 CLIP ( Supplementary Table 6 ). The endogenous expression levels of primary and mature miRNAs were measured via quantitative RT–PCR (qRT–PCR) of U87MG RNA following ADAR1 overexpression (OE) or KD. For miR-21 and miR-34a, ADAR1 OE led to decreased unprocessed pri-miRNA levels and increased mature miRNA expression, whereas ADAR1 KD had the opposite effects ( Fig. 4c ). In contrast, processing of pri-miR-100 was reduced following ADAR1 OE and enhanced in ADAR1 KD cells ( Fig. 4c ). To expand the analysis to the genome-wide scale, we obtained small RNA-sequencing data in U87MG cells transfected with an ADAR1 siRNA, an ADAR1 OE vector or corresponding controls. Consistent with the qRT–PCR results, the expression levels of both miR-21-5p and miR-34a-5p were significantly increased, while that of miR-100-5p was reduced, in cells that express ADAR1 ( Fig. 4d , Supplementary Table 7 ). Overall, if all miRNAs were considered regardless of ADAR1 binding, more miRNAs were observed with enhanced levels associated with ADAR1 expression compared with those with reduced levels ( Supplementary Fig. 12 ). Since these changes could be induced directly or indirectly by ADAR1 function, we further focused on miRNAs interacting with ADAR1 in the CLIP data. For miRNAs bound by ADAR1 in the form of pri-miRNA, we observed a significant bias of enhanced (compared with repressed) mature miRNA levels by ADAR1 expression in both KD and OE samples ( Fig. 4d , Supplementary Fig. 12 ). Notably, there was a significant overlap between miRNAs with pri-miRNA binding by ADAR1 and those with enhanced expression by ADAR1 overexpression ( P =6.7e−04, hypergeometric test). No significant overlap was observed for miRNAs whose expression was repressed by ADAR1 or bound in precursor or mature forms. Together our data suggest that miRNA expression is predominantly enhanced by ADAR1 via its interaction with primary miRNA transcripts. Functional domains of ADAR1 in miRNA biogenesis Since ADAR1 is a dsRBP, it is natural to hypothesize that the impact of ADAR1 on pri-miRNA processing is executed through its binding to the dsRNA structure of the pri-miRNA transcript. To test this hypothesis, we generated an ADAR1 mutant (namely, the EAA mutant) that lost its RNA-binding capability [40] and conducted small RNA sequencing following transfection of this mutant or a control vector to U87MG cells. Compared with the wild-type ADAR1 that showed a global enhancement of miRNA expression, the EAA mutant demonstrated a much less enhancing impact on miRNA levels ( Fig. 4e ). Similarly, we also examined the involvement of ADAR1’s editing activity in miRNA biogenesis using the E912A mutant that has an inactive deaminase domain [29] . Again, this mutant did not enhance miRNA expression to the same extent as the wild-type ADAR1 ( Fig. 4e ). Our data suggest that both RNA binding and RNA-editing activities of ADAR1 likely contribute to the observed impact of this protein in enhancing miRNA biogenesis. ADAR1 associates with both DROSHA and DGCR8 Since it is well established that the microprocessor is required for primary miRNA processing in canonical miRNA biogenesis pathways, we examined whether ADAR1 interacts with DROSHA and/or DGCR8 via the co-immunoprecipitation (Co-IP) experiment ( Fig. 4f , Supplementary Fig. 13 ). Reciprocal Co-IP was conducted using DROSHA, DGCR8 or ADAR1 antibody for IP and immunoblotting (IB), respectively. In the absence of RNase A, all the three proteins were detected with positive Co-IP signals with respect to each other, while the IgG controls were negative. It should be noted that DROSHA is relatively lowly expressed, thus with weak Co-IP signals. In addition, treatment with RNase A (mainly degrading single-stranded RNA (ssRNA)) during the IP step did not alter the results significantly. The observed interactions between DROSHA and DGCR8 (known to be ssRNA independent [41] ) serve as positive controls of the experiment. These data suggest that ADAR1 interacts with the microprocessor reciprocally and that this interaction is not mediated by ssRNA. A general model for the functional roles of ADAR1 A unifying model for the roles of ADAR1 in both 3′ UTR formation and miRNA biogenesis is a binding competition model between ADAR1 and other related proteins ( Fig. 5 ). Our analysis of canonical 3′ UTR processing factors (CF I m 68, CstF64 and CstF64τ) strongly suggests that ADAR1 binding could preclude binding of the other proteins. To provide further evidence, we carried out a cellular fractionation experiment and observed that ADAR1 proteins are predominantly localized in the chromatin fraction in U87MG cells ( Supplementary Fig. 11 ). These data indicate that ADAR1 could occupy nascent RNAs shortly after they were produced, thus rendering an advantage in the competition model. The microprocessor, DROSHA and DCGR8 are relatively enriched in the nucleoplasmic fraction of U87MG cells ( Supplementary Fig. 11 ). Thus, for microRNA processing, the competition model also applies where ADAR1 first occupies (and possibly edits) the nascent pri-miRNA transcripts through recognition of the double-stranded regions and, subsequently, the microprocessor cleaves the substrates. The microprocessor may or may not bind to the RNA in this case, but the pri-miRNA cleavage is enhanced by the presence of ADAR1 ( Fig. 5 ). Figure 5: Schematic models of ADAR1 function in the nucleus on 3′ UTR processing and miRNA biogenesis. These regulatory mechanisms are mainly executed by ADAR1 binding to non- Alu regions. ADAR1 may compete with other cleavage and polyadenylation factors (CF I m 68, CstF64 and CstF64τ) in binding to 3′ UTRs. In the presence of ADAR1, the three proteins impose reduced regulatory influence on ADAR1-bound 3′ UTRs than on other 3′ UTRs. Following ADAR1 KD, these proteins could gain more access to the 3′ UTRs and exert regulation. The proximal cleavage site is often chosen in the presence of ADAR1, whereas the distal site is used on ADAR1 KD. These outcomes reflect combinatorial regulation by the cleavage and polyadenylation factors that have opposing impacts on alternative 3′ UTR usage. For pri-miRNA processing, ADAR1 may bind to (and edit) the nascent primary transcript before DROSHA/DGCR8 binding. The microprocessor then cleaves the pri-miRNA with or without binding to the RNA. The binding of ADAR1 mainly promotes the processing of pri-miRNA, leading to an enhanced miRNA expression level. Full size image The global analyses in this study yielded insights into ADAR1 function and established genomic resources for future functional, mechanistic and modelling studies. With the first genome-wide binding map of ADAR1, highly reproducible binding sites of this protein were identified in >10,000 genes, suggesting a broad target landscape. As a main mediator of A-to-I editing that often occurs in Alu regions in human, ADAR1 was found to bind to numerous Alu repeats across the human genome, which was long expected but never reported globally. A number of novel insights were revealed regarding its involvement in RNA editing, such as a strong structural motif within the right arm of the sense Alu elements, close proximity of the deaminase domain to the RNA and global support for the existence of site-selective and promiscuous editing. These findings will provide a foundation to better understand the selectivity and specificity of editing substrates in future studies. A surprise resulted from our data is the unexpectedly large fraction of ADAR1-binding sites in non- Alu regions. On the basis of this observation, we discovered that the functional significance of ADAR1 is much more diverse than previously appreciated. Examination of ADAR1’s binding to 3′ UTRs, mostly in non- Alu regions, revealed that it is involved in the regulation of alternative 3′ UTR usage. Alternative 3′ UTR usage as a result of APA is emerging as a major player influencing gene expression in animals and plants [42] . This process is closely regulated in development and differentiation and can be dysregulated in disease [43] . Mechanisms mediating APA are just starting to be deciphered. Our study represents the first report that ADAR1 protein is one of the players regulating APA. We found that direct 3′ UTR targets of ADAR1 were lengthened due to usage of distal cleavage sites following ADAR1 KD. Interestingly, these 3′ UTRs were less often regulated by canonical 3′ UTR processing factors, CF I m 68, CstF64 and CstF64τ, compared with controls or shortened 3′ UTRs. A parsimonious model that could explain these observations is that binding of ADAR1 to the 3′ UTRs precluded abundant binding of CF I m 68, CstF64 and CstF64τ ( Fig. 5 ). Consequently, the three proteins impose less regulatory influence on ADAR1-bound 3′ UTRs than on other 3′ UTRs in the presence of ADAR1. The binding profile of ADAR1 in 3′ UTRs ( Fig. 3c ) showed broad peaks encompassing hundreds of nucleotides, which reflects its recognition of dsRNA structures. In contrast, CF I m 68, CstF64 and CstF64τ demonstrated high positional specificity in binding ( Fig. 3d ). Regions with differential ADAR1 binding do not coincide exactly with those with differential binding of the other three proteins. One plausible explanation is that the dsRNA structures are much larger than the ADAR1 footprint captured by CLIP (that is, Fig. 3c ) such that they extend into the otherwise binding sites of the other proteins. A remaining question is whether ADAR1 or its interacting partners can stabilize the underlying RNA structures, which may destabilize (to some extent) following ADAR1 KD and allow release of ssRNA for other proteins to bind. Alternatively, A-to-I editing induced by ADAR1 may stabilize RNA structures [44] . The two mechanisms may both exist, influencing different genes since we observed that the deaminase activity of ADAR1 was necessary to affect 3′ UTR usage of one gene, but not the other ( Fig. 3b ). ADAR family members have been shown to edit a few miRNAs [3] . Editing of pri-miRNA by ADAR1, presumably in the nucleus, could suppress its processing by DROSHA [45] , or inhibit pre-miRNA cleavage by DICER [46] . Thus, in the small number of well-studied examples, the interactions between ADAR1 and pri-miRNAs mainly induced the downregulation of miRNA expression or function. Here our global analysis of the impact of ADAR1 on primary miRNA processing in the nucleus showed that ADAR1 predominantly enhances miRNA expression ( Fig. 4 ). Importantly, our data do not contradict existing literature since the small number of known ADAR1-repressed miRNAs (miR-143 and miR-151 (refs 45 , 46 ) was also suppressed by ADAR1 in our data ( Supplementary Table 7 ; other previously reported miRNAs were lowly expressed in U87MG cells). Thus, our study provides a global, unbiased view of the impact of ADAR1 on pri-miRNA processing, which suggests that the previous literature was not complete. We found that the enhancement of miRNA expression by ADAR1 via its interaction with the pri-miRNAs was generally dependent on both RNA binding and deaminase activities of this protein, although exceptions do exist ( Fig. 4e ). This global result is consistent with the previous literature where editing in pri-miRNAs was necessary to alter processing by DROSHA or DICER [3] . However, it was not clear whether ADAR1 is involved in other aspects of this process beyond RNA editing. Our data confirmed that such additional layers of mechanisms do exist. We showed that ADAR1 interacts with both DGCR8 and DROSHA and the interactions are not dependent on ssRNA substrates ( Fig. 4f ), which is partly consistent with a previous study that showed interaction between ADAR1 and DGCR8 (ref. 47 ). We proposed that ADAR1 binds to nascent pri-miRNA transcripts, likely before the binding by the microprocessor ( Fig. 5 ). For the exact mechanism of ADAR1’s involvement in pri-miRNA processing, two possibilities may exist. One is that RNA editing may alter RNA structure and accessibility of DROSHA to the pri-miRNA transcripts. The second is that the interaction with ADAR1 could enhance/stabilize the microprocessor’s cleavage/binding of the pri-miRNA. Specific pri-miRNA substrate may be subject to one or both of the mechanisms, which will need to be examined on a case-by-case basis. Overall our data suggest that the impact of ADAR1 on pri-miRNA processing in the nucleus may not be limited to RNA editing and the ADAR1-pri-miRNA interaction mainly enhances miRNA expression. Our study complements the previous report that ADAR1 predominantly enhances miRNA production in the cytoplasm in an editing-independent manner [48] . A GO analysis of target genes of ADAR1-affected miRNAs yields a number of categories related to cell proliferation, growth or apoptosis and cellular response to stimuli or DNA damage, among others, ( Supplementary Table 8 ), indicating that this mechanism may have important functional relevance. Recent studies based on RNA-seq data reported numerous A-to-I editing sites in human and other species [49] . However, a vast majority of these editing sites reside in non-coding regions without obvious functional implication. It is known that the embryonic lethality of ADAR1 KO cannot be fully explained by the protein’s function in RNA editing. Possibly, the functional essentiality of ADAR1 roots from its involvement in processes other than RNA editing. Our study provides novel insights for the diverse functional roles of this essential protein and builds a foundation for further mechanistic investigations. Cell culture U87MG cells were purchased from American Type Culture Collection (ATCC). Cells were maintained in DMEM high-glucose medium supplemented with pyruvate, L -glutamine and 10% fetal bovine serum (Gibco, Life Technologies). CLIP-seq CLIP was performed according to previous methods with some modifications [22] , [50] . In brief, U87MG cells were harvested at 90% confluency. Cells were washed once with 10 ml ice-cold PBS. Ultraviolet (254 nm) crosslink 2 × 800 mJ cm −2 was applied with samples on ice. Cell pellets were kept at −80 °C until cell lysis. Cells were lysed in 1 × PBS, 0.1% SDS, 0.5% sodium deoxycholate and 0.5% IGEPAL CA-630. After 30 min lysis on ice, cell lysates were sonicated at 10 s three times with 1-min intervals and then centrifuged at 13,000 g , 4 °C for 10 min. Supernatant was treated with 100 U RNase-free DNase I (Roche) at 37 °C for 30 min and centrifuged at 13,000 g , 4 °C for 10 min. Supernatants were precleared using 50 μl of Dynabeads Protein G (Life Technologies) at 4 °C for 10 min. Hundred μg of ADAR1 antibody (sc-73408 or sc-271854, Santa Cruz Biotechnology) was used for IP at 4 °C overnight. Two hundred μl of Dynabeads Protein G was added and incubated with samples at 4 °C for 4 h on the rotating rocker. Samples were washed twice using lysis buffer and twice with high-salt buffer (5 × PBS, 0.1% SDS, 0.5% sodium deoxycholate and 0.5% IGEPAL CA-630). Subsequently, samples were equilibrated with micrococcal nuclease (MNase) reaction buffer. 20 U of MNase (NEB) was used to treat the samples for 37 °C for 15 min and samples were then washed with the PNK buffer (50 mM Tris-HCl pH 7.4, 10 mM MgCl 2 , and 0.5% IGEPAL CA-630). Calf intestine alkaline phosphatase (50 U) was then applied at 37 °C for 30 min. After three times washing with the PNK buffer, 5 μg of Universal miRNA cloning linker (5′-rAppCTGTAGGCACCATCAAT-NH 2 -3′, NEB) was used as 3′ linker and incubated with 100 U of truncated T4 RNA ligase 2 (NEB) at 22 °C for 4 h. Then RNA was labelled with [γ- 32 P] ATP and samples were run on a 4–12% NuPAGE Bis-Tris gel (Invitrogen). Gel transfer and RNA extraction was carried out following standard CLIP protocol [22] , [50] . 5′ linker ligation was performed at 22 °C for 4 h using 100 pmol of 5′ linker (5′-AGGGAGGACGAUGCGG-3′) and 20 U of T4 RNA ligase (NEB). PCR amplification was run for 23 cycles with 98 °C 10 s, 55 °C 30 s and 72 °C 30 s. PCR products were run on a 4% PAGE gel for size selection (75–250 bp) and purified by phenol extraction. Sequencing libraries were prepared using the Encore NGS library kit (NuGEN) and sequenced on an Illumina HiSeq 2500 sequencer at the UCLA Clinical Microarray Core. Small RNA sequencing U87MG cells were cultured as described above. To perturb ADAR1 expression level, the cells were transfected with one of the following: (1) siRNA of ADAR1 (with sense sequence: 5′-CGCAGAGUUCCUCACCUGUATT-3′) [21] , (2) a scrambled siRNA as control (D-001210-02-05, Dharmacon RNAi Tech), (3) expression vector of wild-type ADAR1, (4) expression vector of ADAR1 EAA mutant, (5) a control vector (pcDNA4, Invitrogen). After 36 h transfection, total RNA was isolated using QIAzol. Spike-in controls (Exiqon) were added at a level of one reaction volume per one μg of total RNA. Small RNAs were isolated using miRNeasy mini kit (Qiagen). Small RNA-sequencing libraries were generated using Illumina TruSeq Small RNA library prep kit according to the manufacturer’s instruction. RNA immunoprecipitation (RIP)-PCR IP was carried out similarly as described in the CLIP experiment. In brief, 90% confluent U87MG cells in the 10-cm plate were harvested and lysed. A total of 10 μg of ADAR1 antibody or anti-mouse IgG (as control) were used for IP (Santa Cruz Biotechnology). Following IP, RNA was isolated using the Trizol approach (Life Technologies). Subsequently, complementary DNA (cDNA) was made by SuperScript III (Life Technologies) using random primers and PCR was carried out for 20 cycles with 98 °C 15 s, 55 °C 15 s and 72 °C 30 s. PCR primers are listed in Supplementary Table 2 for LINE-1, AluY, AluJ, 7SK. β-actin was used as control. PCR products were run on a 4% PAGE gel at 70 V for 1 h and stained with SYBR Green gel staining solution (Lonza). ADAR1 overexpression vectors ADAR1p150 cDNA was cloned into the pEGFP-C1 or pcDNA4-TO-FLAG-myc-His vectors (Invitrogen) using the Not I- Xba I restriction sites (NEB). Two ADADR1p150 mutants, the EAA and E912A mutants, were amplified using Q5 High-Fidelity DNA polymerase followed by Dpn I (NEB) treatment at 37 °C for 1 h (NEB) and transformed into competent DH5α. ADAR1 mutants were also cloned into the pcDNA4-TO-FLAG-myc-His vector as described previously [29] , [40] . All constructs were sequenced and ADAR1 overexpression was confirmed by western blot. PCR primers and the site directed mutagenesis oligos are listed in Supplementary Table 2 . Pri-miRNA and miRNA expression analysis U87MG cells were transfected with 250 ng pcDNA4-TO-FLAG-myc-His (V) or pcDNA4-TO-FLAG-myc-His-ADAR1 (WT), or pcDNA4-TO-FLAG-myc-His-EAA-ADAR1 (EAA), or pcDNA4-TO-FLAG-myc-His-E912A-ADAR1 (E912A) using Effectene transfection reagent (Qiagen) following the manufacturer’s instructions. Scrambled control siRNA or siRNA specific to ADAR1 was transfected, respectively, using RNAiMax (Invitrogen) with 400 pM per six wells according to the manufacturer’s protocol. Sequence of siRNA to ADAR1 is 5′-CGCAGAGUUCCUCACCUGUAU-3′ (ref. 21 ). RNAs from U87MG cells were extracted using TRIzol reagent (Invitrogen). A total of 5 μg RNA was used for reverse transcription by ProtoScript II Reverse Transcriptase (NEB) in a 20-μl volume reaction. Real-time qPCR was run on a Roche LightCycler 480 with a mixture containing 1 μl cDNA, 10 μl LightCycler 480 SYBR Green I Master (Roche) and 250 nM of each primer ( Supplementary Table 2 ). qPCR was performed by denaturing at 95 °C for 5 min, followed by 45 cycles of denaturation at 95 °C, annealing at 60 °C and extension at 72 °C for 10 s, respectively. Co-immunoprecipitation Ten million HeLa cells were lysed by 1 ml non-denaturing lysis buffer (20 mM Tris-HCl pH 8, 137 mM NaCl, 1% Nonidet P-40, 2 mM EDTA) with complete protease inhibitor cocktail. Co-IP experiments were performed using 10 μg ADAR1 antibody (D-8, Santa Crutz, sc-271854), 10 μg DROSHA antibody (Abcam, ab12286) or 2 μg DGCR8 antibody (Abcam, ab90579), or corresponding isotype IgG with Dynabeads Protein G (Life Technology) at 4 °C overnight. Then Protein G-antibody–antigen complex was washed by wash buffer (10 mM Tris, pH 7.4, 1 mM EDTA, 1 mM EGTA, pH 8.0, 150 mM NaCl, 1% Triton-X-100) with complete protease inhibitor cocktail. Protein complex was finally eluted from the Dynabeads using elute buffer (0.2 M glycine, pH 2.8). IP was validated by IB using ADAR1 antibody (15.8.6, Santa Crutz, sc-73408, 1:1,000 dilution), DROSHA antibody (Abcam, ab12286, 1:500 dilution) and DGCR8 antibody (Abcam, ab90579, 1:1,000 dilution) to IB the corresponding antigens. RNase A was used to degrade single-stranded RNA at 20 μg ml −1 for 1 h at 4 °C during antigen–antibody incubation. See Supplementary Fig. 13 for uncropped IB images. Cellular fractionation U87MG cells were fractionated following a previously published protocol [51] with some modifications. In brief, 5 × 10 6 U87MG cells were treated with the plasma membrane lysis buffer (10 mM Tris-HCl, pH 7.5, 0.1% NP-40, 150 mM NaCl) on ice for 4 min. After centrifugation, the supernatant was kept as cytoplasm fraction and the pellet was then treated with nuclei lysis buffer (10 mM HEPES, pH 7.6, 1 mM DTT, 7.5 mM MgCl 2 , 0.2 mM EDTA, 0.3 M NaCl, 1 M Urea, 1% NP-40) after washing. The nucleoplasm and chromatin fraction were then separated by centrifugation. Fractionation efficiency was validated by western blotting using antibody specific to the marker for each fraction: β-tubulin (Sigma, T8328, 1:2,000 dilution) for cytoplasm, rabbit polyclonal U1-70k (a kind gift from Dr Douglas Black, 1:4,000 dilution) for nucleoplasm and Histone 3 (Abcam, ab1791, 1:2,500 dilution) for chromatin. Validation of alternative 3′UTR usage U87MG cells in a 10-cm plate were treated with control or ADAR1 siRNA as in our previous study [21] . After 36 h, RNA was isolated using Trizol (Life Technologies), followed by Direct-zol RNA mini prep kit (Zymo Research). cDNA was made using SuperScript III (Life Technologies) and oligo-dT primer. Real-time PCR was performed using the SYBR Green I Master mix for 40 cycles with 98 °C 10 s, 55 °C 10 s and 72 °C 30 s on a Lightcycler 480 machine (Roche). PCR primers are listed in Supplementary Table 2 . CLIP-seq read mapping Adapter sequences were trimmed from both ends of the raw CLIP-seq reads using cutadapt ( https://code.google.com/p/cutadapt/ , v1.1). The 5′ and 3′ end adapter sequences were examined to determine the strand of the read relative to its corresponding RNA. Reads shorter than 15 nt after adapter trimming were discarded. Subsequently, the reads were mapped to the reference sequences (see below) using Novoalign ( http://www.novocraft.com/main/index.php , v2.08.02) that allows microinsertions and deletions with relatively high accuracy. The alignment parameters were: ‘-o FullNW –t 150 –R 99 –r All –F STDFQ –o SAM’. A step-wise mapping procedure was applied. (1) Reads that aligned to the rRNA sequences (downloaded from UCSC genome browser) were discarded. (2) Reads passing the rRNA filter were aligned to the Alu sequences located in RefSeq genes. This procedure was necessary as a large number of reads were mapped to Alus given the binding preference of ADAR1. (3) Reads that did not map to Alu sequences in (2) were aligned to the whole genome (hg19). (4) Alignment results from (2) and (3) were filtered based on the number of mismatches (7% of each read length after adapter-trimming) and merged. Thus far, the paired-end reads were treated as two single-end reads. (5) The paired-end reads were examined for their concordance by considering the corresponding mapped chromosome, mapped strand, and the distance between the pair of reads. Since Alu sequences are highly similar to each other, we retained the top 10 alignment pairs (based on the number of mismatches in a pair) for each pair of reads. Generation of binding clusters based on CLIP-seq reads Mapped reads were classified as sense- and antisense reads based on the strand of the reads and RefSeq annotations. Only sense reads were used to define binding clusters. In each data set, we removed duplicate reads and kept the one with the least mismatches. To define read clusters as ADAR1-binding sites, we used a strategy similar to that in previous studies [24] , [52] . In brief, the reads were retained for further analysis if they overlapped with pre-mRNAs annotated by RefSeq. A sliding window (83 nt) was applied to determine whether the number of reads in the window exceeded expected values based on both a local and global read frequency. A Poisson model was used to test the significance of read enrichment in each window. The local frequency, specific for each gene, was calculated as the number of reads overlapping that gene divided by gene length. The global frequency was defined for all transcripts in the genome. A Bonferroni-corrected P value cutoff of 0.001 was applied to call significant clusters. The final clusters were classified as Alu and non- Alu clusters based on the annotations from UCSC genome browser repeat track ( http://hgdownload.cse.ucsc.edu/goldenPath/hg19/database/ ). The stringent set of binding clusters was defined as those common to both ADAR1 CLIP experiments. To remove the possible non-protein-specific CLIP artifacts, we further filtered all clusters by removing those common to at least two other public CLIP data sets. Binding preference within Alu consensus Final mapped reads (based on the procedures described above) were used for the analysis of binding preference within Alu elements. Alu consensus sequence was downloaded from Repbase [53] ( http://www.girinst.org/repbase/ ). Reads were realigned directly against the sense and antisense Alu consensus sequences using BLASTN with the parameter ‘-strand plus’. The alignment results were parsed and read enrichment within the consensus sequences was calculated by counting the mapped reads in each position of the sense- or antisense- Alu . As controls, we simulated random reads from all Alu regions mapped by CLIP-seq reads. The simulated read length was 83 bp with 0 mismatches to the genome and the read quality scores were randomly sampled from the CLIP-seq reads. The simulated reads were mapped to the genome in the same way as for the CLIP-seq reads (see the section ‘CLIP-seq read mapping’). Following the mapping process, the final mapped simulated reads were collected and directly realigned against the sense and antisense Alu consensus sequences as described above. For simulated reads mapped to the consensus sequence, we calculated the average density level per base in the sense and antisense Alu region. For each position of the sense and antisense Alu , a normalization factor was then computed by dividing the average density by the current density level at the position. For CLIP-seq reads enrichment in the consensus sequence, normalized read counts were calculated by multiplying the normalization factor. Motif analysis Motif analysis was carried out similarly as described in ref. 21 . In brief, to find enriched sequence motifs in the ADAR1-bound Alu clusters, we first ranked the stringent set of clusters (defined above) based on the average number of mapped reads per position. We collected the top 500 Alu clusters after ranking and searched for motifs using the Multiple Em for Motif Elicitation method [54] . For background control, we used a second-order Markov model generated from random Alu repeat regions. The most significant motif had an E-value of 3.4e−6473 and the motif was detected in 314 out of the 500 clusters. Genome-wide correlation of CLIP density across samples Publicly available data of protein–RNA interactions were examined for hnRNP A1, A2/B1, F, M, U (GSE34996) [55] , hnRNP H (GSE23694) [56] and hnRNP C (GSE25681) [57] . Using these data and the two ADAR1 CLIP data sets in this study, the correlation of CLIP density between any two samples was determined similarly as described in ref. 58 . In brief, CLIP tags in 3′ UTRs were analysed for highly expressed genes with high CLIP coverage (>100 tags per UTR). Pearson correlation coefficients were computed between each pair of samples/proteins. Analysis of crosslinking-induced errors in CLIP-seq reads It is known that CLIP reads may include one or more mutations that correspond to the crosslinking sites between the protein and the RNA [28] . To determine which type of mutation reflects the crosslinking sites, we compared the profiles of substitutions, deletions and insertions in the actual CLIP reads to those in simulated reads for both ADAR1 antibodies ( Supplementary Fig. 6 ). For each read position, the frequency of observing a specific type of mutation is calculated by comparing read sequences to the reference genome of U87MG. Simulated reads were generated by extracting short-read sequences from the reference genome and with simulated read quality scores mimicking those of actual reads. Simulated reads were mapped in the exact same way as for the actual reads. As shown in Supplementary Fig. 6 , deletion errors were significantly more prevalent (roughly 10-fold higher) in CLIP-seq reads than in simulated reads and the deletion frequency is relatively high near the centre of the reads. This observation holds for the CLIP-seq libraries generated by both antibodies and for reads mapped to both Alu and non- Alu regions. Thus, deletion in CLIP-seq reads is a useful feature related to crosslinking sites. Distance between ADAR1 CLIP sites and RNA-editing sites To check whether the editing sites are close to the binding sites of ADAR1, the shortest distance between A-to-I editing sites (from DARNED database, http://darned.ucc.ie/ [34] ) and the CLIP clusters was calculated by taking the minimum difference between the coordinates of editing sites and starting or ending positions of the cluster in a gene. Three different distances were computed: (1) linear distance: linear genomic distance, (2) structural distance: distance calculated between predicted dsRNA structures harbouring CLIP clusters and editing sites and (3) control distance: distance between CLIP clusters and random A’s in the same gene. For the calculation of structural distance, we generated all pair-wise alignments between CLIP clusters and Alu elements in the same gene using a BLAST-like algorithm (unpublished). Within a predicted structure, both CLIP clusters and the associated Alu elements were considered to get the minimum distance between the cluster and the editing sites. Conservation analysis of regions flanking editing sites The same method as in our previous work [21] was used to evaluate the conservation level of each editing site and their flanking regions. In brief, with the 46-way multiz alignments from the UCSC browser [59] , we focused on the 10 primates among these 46 species, including Human, Chimp, Gorilla, Orangutan, Rhesus, Baboon, Marmoset, Tarsier, Mouse lemur and Bushbaby. On the basis of the multiple sequence alignments, the per cent identity at each nucleotide position of interest was calculated. CLIP-seq analysis for miRNA binding Genomic coordinates of human miRNAs and precursors were downloaded from miRBase (Release 19). CLIP-seq reads were examined to retain those located within or less than 100 nt from the pre-miRNAs. The read pileup for each miRNA region was analysed to determine whether there were patterns representing ADAR1 binding to mature, pre- or pri-miRNA. Specifically, binding to mature or pre-miRNA was required to be associated with read distributions following a boxcar function. A minimum of five reads was required. The boundaries of the boxcar distribution (and the start and end of all reads) were not allowed to vary from the annotated start and end of the mature or pre-miRNA by more than two nucleotides. Note that certain reads matching the mature form of miRNAs could have originated from digested pre-miRNA or pri-miRNA transcripts during CLIP library preparation. Similarly, pre-miRNA-matching reads could have originated from digested pri-miRNAs. However, it is unlikely that such random digestions result in a pileup of CLIP tags with similar start and end positions. Thus, we evaluated the significance of the uniformity of CLIP tag start/end positions matching the mature or pre-miRNA isoforms against a background distribution assuming random start/end locations. A P value cutoff of 0.05 was applied to define whether a group of CLIP tags represented the mature or pre-miRNA forms. To call positive binding to pri-miRNA, a minimum of five reads was required to map within 100 nt of the pre-miRNA and at least one read should overlap with the pre-miRNA. CLIP-seq data generated using the two ADAR1 antibodies were analysed separately. The final list of ADAR1-bound mature, pre- and pri-miRNAs consists of a union of the two sets of results. Small RNA-seq data analysis Small RNA-seq reads were first processed to remove adapter sequences and low-quality reads. The reads were then aligned to the human genome using Bowtie [60] allowing at most one mismatch. The mapping results were parsed to identify reads mapped to miRNAs (miRBase, Release 19). Only reads mapped uniquely to the miRNAs were retained. In parallel, reads were also aligned to the spike-in controls allowing no mismatches. The number of reads mapped to each miRNA was normalized using the spike-in controls and total number of mapped reads in each library. The abundance of spike-in RNA was highly correlated across libraries. Using the spike-in data, a log fold-change (LFC) cutoff was determined at a false discovery rate of 5% for each pair of libraries (si-ADAR1 versus si-control, wt-ADAR1 versus control, EAA versus control). Differentially expressed miRNAs across each pair of libraries were then identified as those with LFC no less than the above cutoff and at least 16 reads in at least one library. RNA-seq data analysis for alternative 3′ UTRs For annotated genes (RefSeq), we developed a new method to identify the core and extension regions of tandem 3′ UTRs using RNA-seq data alone without relying on annotation of alternative 3′ UTRs. Specifically, we assume the RNA-seq read counts follow a multivariate mixture normal distribution with two components representing the core and extension regions of the 3′ UTR. Read counts of each nucleotide in the candidate 3′ UTR was represented by the two components and the goodness-of-fit of the model was estimated using Bayesian information criterion (BIC). The predicted core and extension regions were required to be associated with the highest BIC value. Since many 3′ UTRs may not have alternative cleavage sites, we also calculated the BIC value of the model with only one component (no core/extension boundary in the 3′ UTR), and compared it with the maximum BIC of the two-component model. If the BIC from the two-component model is larger than that from the one-component model, we will consider this 3′ UTR as an alternatively processed 3′ UTR. To elucidate the influence of ADAR1 on 3′ UTRs, we calculated the relative change (RC) of read coverage of the extension region and that of the core region between the ADAR1 KD and controls samples. That is, RC =log 2( ext KD / ext control )−log 2( core KD / core control ). where, ext KD and ext control represent the mean of read coverage of extension region in ADAR1 KD and control samples, respectively; similarly for core KD and core control . We retained 3′ UTRs with |RC|≥0.5 as candidates that are impacted by ADAR1, with the other 3′ UTRs as controls. A P value-based filter was not further applied to get a relatively large number of 3′ UTRs (thus statistical power) for further analyses. This choice of cutoff parameters represents a trade-off between statistical power and across-group difference. GO analysis GO analysis was conducted similarly as in ref. 61 . In brief, the GO terms of each gene were obtained from Ensembl. To identify GO categories that are enriched in a specific set of genes, the number of genes in the set with a particular GO term was compared with that in a control gene set. The control gene set was constructed so that the randomly picked controls and the test genes have one-to-one matched transcript length and GC content. On the basis of 10,000 randomly selected control sets, a P value for the enrichment of each GO category in the test gene set was calculated as the fraction of times that F test was lower than or equal to F control , where F test and F control denote, respectively, the fraction of genes in the test set or a random control set associated with the current GO category. A P value cutoff (1/total number of GO terms considered) was applied to choose significantly enriched GO terms. Accession codes: The high-throughput sequencing data have been deposited in Gene Expression Omnibus under the accession code GSE55363. How to cite this article: Bahn, J. H. et al. Genomic analysis of ADAR1 binding and its involvement in multiple RNA processing pathways. Nat. Commun. 6:6355 doi: 10.1038/ncomms7355 (2015).